Spatial optimization of carbon-stocking projects across Africa integrating stocking potential with co-benefits and feasibility Carbon offset projects through forestation are employed within the emissions trading framework to store carbon. Yet, information about the potential of landscapes to stock carbon, essential to the design of offset projects, is often lacking. Here, based on data on vegetation carbon, climate and soil, we quantify the potential for carbon storage in woody vegetation across tropical Africa. The ability of offset projects to produce co-benefits for ecosystems and people is then quantified. When co-benefits such as biodiversity conservation are considered, the top-ranked sites are sometimes different to sites selected purely for their carbon-stocking potential, although they still possess up to 92% of the latter carbon-stocking potential. This work provides the first continental-scale assessment of which areas may provide the greatest direct and indirect benefits from carbon storage reforestation projects at the smallest costs and risks, providing crucial information for prioritization of investments in carbon storage projects. The primary aim of carbon (C)-stocking projects is to reduce atmospheric C concentrations to mitigate anthropogenic climate change; therefore, a central component in feasibility assessments of C-stocking projects is their potential to store C ( [1] ). Storing C in vegetation constitutes an important focus for C-stocking projects because human land-use often results in vegetation C storage that is less than its potential maximal value under prevailing environmental conditions. Notably, forest degradation due to logging, grazing and fuel wood collection, or deforestation from conversion of forests to agricultural land, may result in decreases in C storage, with forest C sinks converted to C sources [2] , [3] . Deforestation is the second largest source (15%) of greenhouse gas release into the atmosphere, a trend that is expected to continue due to human population increases and ongoing land-use changes, while climate change may lead to additional forest losses and release of greenhouse gases [4] , [5] , [6] . Other natural and anthropogenic disturbances such as herbivory [2] and more frequent or intense fires [3] may also decrease vegetation C storage. Understanding the difference between potential and actual C storage is therefore essential for assessing the scope for C stocking in vegetation. While vegetation C-stocking projects focus on reducing atmospheric C concentrations, they may have secondary benefits for biodiversity, ecosystem services and local economies. For example, C-stocking projects can provide payments to the local communities in which they are based [7] . Biodiversity conservation can also be promoted through, for example, habitat restoration [8] or conservation of species [9] , and reforestation and restoration of degraded vegetation can contribute to ecosystem services like water flow regulation, soil protection, flood regulation and the provision of food and other non-timber forest products [9] , [10] . Such co-benefits are often overlooked when establishing C-stocking projects [11] . In fact, in the voluntary market, 40% of forest C projects use exotic species [12] . Since many C-stocking projects constitute monocultures and may involve the transformation of natural grasslands to exotic plantations, they can harm biodiversity and other ecosystem services [9] . While monocultures of fast-growing species can have the advantage of rapidly storing significant amounts of C, they may cause problems such as altering water supply and driving species loss, and some exotic plantation species can become invasive, with further-reaching ecological and economic consequences [13] . In summary, it is advantageous to consider biodiversity and other ecosystem co-benefits in C forest projects not only to avoid unintended adverse effects but also to ensure sustainability of such projects by enhancing their value to local people and attracting more and diverse potential investors [14] . Within the developing world, Africa is under-represented in terms of forest-based C-stocking projects and projects in Africa tend to be geographically biased, with the majority located in East Africa [9] . However, Africa is one of the fastest growing regions for the voluntary C market, with much of the growth driven by consumer demand for projects geared towards sustainability [15] . Many of the recent C projects in Africa have been certified by high-quality standards [15] , which, among others, assess carbon storage, audit projects, ensure transparency and evaluate multiple benefits of carbon projects. Given these positive trends, and the apparent demand in the C market for benefits other than C storage, Africa holds promise for further and more integrated C-stocking projects. Yet, for C-stocking projects that have been initiated in Africa, information on the ability of landscapes to stock C has often been missing before project initiation [9] . To ensure the long-term sustainability of these projects and to provide the desired returns, it is crucial to establish more systematic identification of the areas with the potential to store significant amounts of C, while also considering their potential co-benefits. Recent advances in data availability have made such systematic approaches feasible. For example, aboveground C storage has been quantified across broad spatial scales using remote sensing, enabling the generation of maps of aboveground C storage for continental regions [16] , [17] . These broad-scale maps, coupled with an understanding of the factors that affect vegetation C storage, can be used to estimate the potential of regions to store C by means of forestation programmes. In addition, spatial prioritization techniques developed for systematic conservation planning provide powerful tools for choosing sites that offer the best solutions to multiple criteria such as co-benefits and costs. Here, to help guide international investments in C storage, we develop and test such a systematic approach to the prioritization of investments in C storage projects across tropical Africa. We quantify the potential for aboveground C stocking in forests in the absence of human disturbance for tropical Africa to identify where C stocking through forestation might provide the greatest benefits. A spatial prioritization technique is subsequently employed to identify areas where C-stocking projects could also provide other benefits and reduce costs. Generation of maps showing potential for C stocking Maps of C-stocking potential, that is, additional C that could be stored in vegetation if disturbances were eliminated, were produced for tropical Africa. Different C-stocking potential maps were produced based on two available maps of aboveground C storage: that by Saatchi et al. [16] and Baccini et al. [17] ( Fig. 1 , Supplementary Fig. S1 , Supplementary Table S1 ). We also employed two different modelling methods, 90% quantile regression (QR) and ordinary least square (OLS) regression analyses, to generate maximum C biomass maps, which were used to produce the C-stocking potential maps. The coefficients of the QR and OLS models are presented in Supplementary Table S2 . These coefficients were similar to coefficients produced from 2,000 set of analyses that were run on random subsets of the data set, for both Saatchi- and Baccini-produced maximum C biomass maps, although confidence was higher for the former than the latter ( Supplementary Tables S2 and S3 ). A map of model uncertainty per planning unit (PU) for maximum C biomass is given in Supplementary Fig. S2 . There was geographic variation in uncertainties between areas, but variation in estimates remained small, indicating low uncertainty. We also evaluated how well the predicted maximum C biomass corresponded to actual values of C biomass in undisturbed forests. There was a positive relationship between the two (except for the 98% QR maps based on the Saatchi data set, Supplementary Table S4 and Supplementary Fig. S3 ). The r 2 -values between the field data and the predicted C biomass were not much different from those between the field data and the original C biomass maps, although the latter had slopes closer to one ( Supplementary Table S4 , Supplementary Fig. S3 ). The Baccini-generated maximum C biomass map better matched the field data than that of the Saatchi map did ( Supplementary Table S4 , Supplementary Fig. S3 ). Nevertheless, due to the above-mentioned higher confidence in the Saatchi data set, and because the two original maps by Saatchi and Baccini are highly correlated for the study area (87%, Supplementary Table S5 ), we focus on the analyses based on the more recently produced Saatchi data set, although most analyses were repeated on the Baccini-based data ( Supplementary Figs S1, S4 and S5 ). Carbon-stocking potential maps produced by QR and OLS analyses were highly correlated (>92%, Supplementary Table S5 ). For this reason, and because the human influence index [18] on which the OLS analyses were based ( Supplementary Methods ) may not be an altogether accurate measure of vegetation degradation [18] , we here report the results from the QR analysis, while OLS results are presented in Supplementary Figs S1, S4 and S5 . 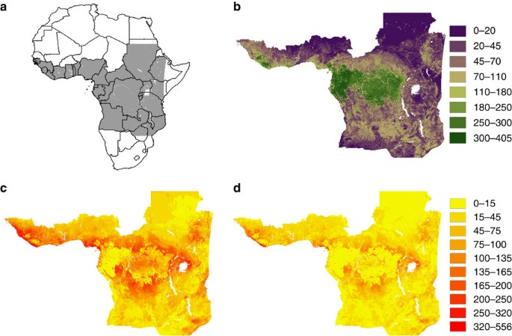Figure 1: Saatchi carbon maps. (a) Map of extent of study area. (b) Woody biomass (mapped from16) and C-stocking potential (the difference between the potential woody biomass and the actual woody biomass) as calculated by (c) 90% quantile regressions and (d) ordinary least square regressions with human influence set to zero. Carbon values were taken from Saatchiet al.16 Figure 1: Saatchi carbon maps. ( a ) Map of extent of study area. ( b ) Woody biomass (mapped from [16] ) and C-stocking potential (the difference between the potential woody biomass and the actual woody biomass) as calculated by ( c ) 90% quantile regressions and ( d ) ordinary least square regressions with human influence set to zero. Carbon values were taken from Saatchi et al. [16] Full size image The areas with the greatest C-stocking potential were the western Upper Guinean rainforest, the Lower Guinean rainforest (both particularly predicted by the computations based on the Saatchi map, Fig. 1 ), pockets north and south of the Congolian rainforests and the area around Lake Victoria (especially predicted by the computations based on the Baccini map) ( Figs 1 , 2 and Supplementary Fig. S4f ). In contrast, the Congolian rainforests (for the Saatchi data only the western sections) and the Sahel exhibited low levels of C-stocking potential. The total additional woody biomass that could be stored in vegetation across the entire region amounted to 8.90 × 10 10 T (based on 90% QR analyses conducted on the Saatchi C map; Fig. 1c ). The total additional woody biomass that could be stored in vegetation across the entire region amounted to 1.06 × 10 11 T when C storage was calculated using 90% QR models based on the Baccini C map, and 3.93 × 10 10 T or 4.40 × 10 10 T when C storage was calculated using OLS models based on the Saatchi and Baccini C maps, respectively. 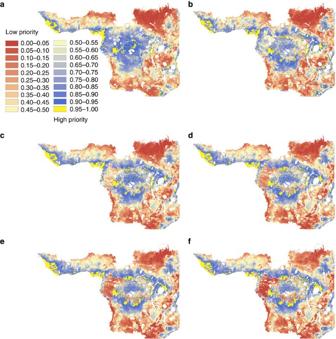Figure 2: Priority rank maps of tropical Africa based on quantile regression C maps. Priority rank maps based on Zonation analyses, showing the areas that would be most suitable for carbon sequestration projects while also benefitting biodiversity, groundwater recharge, land value and governance. Maps (a–e) represent different analyses, where the weighting of C-stocking potential was altered between 3 (a), 6 (b), 12 (c), 24 (d) and 48 (e), while the weight of all other features was kept constant at 12. Map (f) represents the carbon only map, which was generated using C-stocking potential alone and did not consider any other benefits or costs; it is thus a ranking of sites in terms of the C-stocking potential. Yellow areas indicate the 5% highest-ranked planning units and are thus deemed high priority, whereas red areas indicate the lowest-ranked planning units and are deemed low priority. Carbon-stocking potential was calculated from the Saatchi map using 90% quantile regressions. The ABF cell removal rule was used in Zonation analyses. Figure 2: Priority rank maps of tropical Africa based on quantile regression C maps. Priority rank maps based on Zonation analyses, showing the areas that would be most suitable for carbon sequestration projects while also benefitting biodiversity, groundwater recharge, land value and governance. Maps ( a – e ) represent different analyses, where the weighting of C-stocking potential was altered between 3 ( a ), 6 ( b ), 12 ( c ), 24 ( d ) and 48 ( e ), while the weight of all other features was kept constant at 12. Map ( f ) represents the carbon only map, which was generated using C-stocking potential alone and did not consider any other benefits or costs; it is thus a ranking of sites in terms of the C-stocking potential. Yellow areas indicate the 5% highest-ranked planning units and are thus deemed high priority, whereas red areas indicate the lowest-ranked planning units and are deemed low priority. Carbon-stocking potential was calculated from the Saatchi map using 90% quantile regressions. The ABF cell removal rule was used in Zonation analyses. Full size image For some PUs, the C-stocking potential exceeded the maximum C storage values given in the original C biomass maps obtained from Saatchi et al. [16] and Baccini et al. [17] . We do not propose that the potential C-stocking values we obtained are absolute values—they are more likely to provide indications of relative values. In contrast, there are indications that the maximum C biomass for Africa that is provided by both original C biomass maps are actually surpassed in the tropical forests of Africa [19] , [20] , [21] (for example, 596 T x ha-1, recorded in Cameroon [19] ), indicating that it is not impossible that there are regions with the higher C-stocking potential values we obtained in our models. Therefore, the C-stocking potential values should be interpreted more as relative rather than absolute values. Identifying where C-stocking projects can have co-benefits Next, we assessed which PUs not only possess high C-stocking potential but would also hold co-benefits and have lower costs associated with them. When biodiversity measures, groundwater recharge and socioeconomic factors were considered along with C-stocking potential to select PUs for C stocking ( Fig. 2 , Supplementary Fig. S4a–e ), the top 5% highest-ranked PUs differed from those ranked only by their C-stocking potential ( Fig. 2 , Supplementary Fig. S4f ), except when C-stocking potential in the multi-criteria selections was weighted particularly high with respect to the other features, resulting in similar prioritizations. This indicates that the PUs identified as most suitable for C stocking were not always most beneficial in terms of co-benefits, costs and risks ( Fig. 2 , Supplementary Fig. S4a–e versus S4f ). The distribution of high-ranking PUs also differed depending on the cell removal rule used ( Supplementary Fig. S4 , ‘added benefit function (ABF)’ versus ‘basic core zonation (BCZ)’ method). The ranking of PUs differed between runs with different weightings for C-stocking potential ( Fig. 2 ). Although similar contiguous areas with a concentration of highly ranked PUs were usually identified in analyses with different C-stocking potential weightings, their size and extent changed as the importance of C-stocking potential varied ( Fig. 3 , Supplementary Fig. S5 ). As the weighting of C-stocking potential decreased, and the other factors thus gained in importance, there were fewer highly ranked sites around Lake Victoria and north and south of the Congolian rainforests (with the exception of the Batéké Plateau), while there was an increasing concentration of highly ranked sites in the Lower Guinean rainforests. As expected, runs with more similar weightings of C-stocking potential showed more overlap in the top 5% rankings of PUs ( Supplementary Table S6 ) and showed less change in overall rankings ( Supplementary Table S7 ) than runs with more dissimilar rankings. 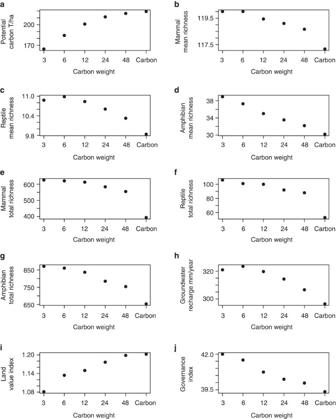Figure 3: Performance plots at different weightings of C-stocking potential weightings. The performance of the 5% top-ranked planning units (yellow areas inFig. 2) when the C-stocking potential was differently weighted (3, 6, 12, 24, 48, Carbon only; x-axis) in Zonation analyses is shown. (a) ‘Potential Carbon’—the total additional C biomass that could be stored in all 5% top-ranked planning units. (b–d) Biodiversity ‘Mean Richness’—the mean richness per 5% top-ranked planning unit. (e–g) Biodiversity ‘Total Richness’—the taxon richness summed across all 5% top-ranked planning units. (h) Groundwater recharge, (i) land-use value and (j) governance were averaged across all 5% top-ranked planning units in the landscape. The C-stocking potential map was generated by 90% QR on the Saatchi data set, and the ABF cell removal rule was used in Zonation analyses. Figure 3: Performance plots at different weightings of C-stocking potential weightings. The performance of the 5% top-ranked planning units (yellow areas in Fig. 2 ) when the C-stocking potential was differently weighted (3, 6, 12, 24, 48, Carbon only; x-axis) in Zonation analyses is shown. ( a ) ‘Potential Carbon’—the total additional C biomass that could be stored in all 5% top-ranked planning units. ( b – d ) Biodiversity ‘Mean Richness’—the mean richness per 5% top-ranked planning unit. ( e – g ) Biodiversity ‘Total Richness’—the taxon richness summed across all 5% top-ranked planning units. ( h ) Groundwater recharge, ( i ) land-use value and ( j ) governance were averaged across all 5% top-ranked planning units in the landscape. The C-stocking potential map was generated by 90% QR on the Saatchi data set, and the ABF cell removal rule was used in Zonation analyses. Full size image As the weighting of C-stocking potential increased in Zonation analyses, the C-stocking potential of the highest ranked sites increased ( Fig. 3 and Supplementary Fig. S5a–e ), while the performance of ecosystem services and economic risks and costs suffered reductions ( Fig. 3 , see also Supplementary Fig. S5 ). The performance of features showed more consistent trends for all features when the ABF, rather than the BCZ, cell removal rule was used. The performance of the various features was erratic for analyses conducted using BCZ. For example, for the 90% QR analyses based on the Saatchi data the performance potential C stored was lower for analyses weighted 12 than 6 ( Supplementary Fig. S5 ), although one would have expected the reverse pattern. Therefore, our interpretations were entirely based on analyses conducted using the ABF cell removal rule. For ABF analyses, benefits other than C-stocking potential predictably decreased and penalties increased with increasing C-stocking potential weightings ( Fig. 3 and Supplementary Fig. S5a–e ). (Only the effects of increasing the C-stocking potential weighting on biodiversity were somewhat dependent on whether species richness was averaged per PU or summed across the entire landscape ( Fig. 3 ). Species richness summed across the landscape performed as expected—it tended to decrease with increasing C-stocking potential, while mean species richness per PU did not always show consistent trends. This is because species richness summed across the landscape better represents the conservation objectives of the site selection method used here: highly ranked sites should support different subsets of species rather than purely harbour high species richness.). Since the primary aim of this study was to identify regions with potential for C stocking that would also, secondarily, benefit ecosystem services at minimal socioeconomic cost and risk, we focused on the ranking of PUs in which C-stocking potential was assigned the sum of the weights of all other factors, that is, 12 ( Fig. 2c ). This strategy ensured that C-stocking potential was neither down-weighted by, nor dominant over, the other features in the PU selection process. Indeed, the amount of C that could be stored in the 5% highest-ranked PUs of this procedure (90% QR Saatchi ABF analyses) was 92% of that of the 5% highest-ranked PUs based on C-stocking potential only, while total mammal, reptile and amphibian species richness were 56, 89 and 28% higher, respectively; groundwater recharge and governance were 8 and 3% higher, respectively, and total land value 5% lower than if sites had been chosen based on C-stocking potential only ( Fig. 3 ). (See Supplementary Fig. S5 for results of other analyses). Three large contiguous areas emerged as having high C-stocking potential and co-benefits ( Fig. 2c , yellow areas): the Upper and Lower Guinean Forests and the Batéké Plateau. As mentioned, other regions surrounding the Congolian rainforests and the areas around Lake Victoria showed high potential for C-stocking alone but did not perform as strongly when other factors were taken into consideration ( Fig. 2 , Supplementary Fig. S4 ). Connectivity parameters were included and varied to identify larger contiguous areas of high ranking during the site selection process ( Supplementary Fig. S6 ). As expected, the larger the connectivity parameter used, the larger were the contiguous patches of highly ranked PUs ( Supplementary Fig. S6 ), although the total C-stocking potential and other benefits in the top-ranked sites generally decreased, with some variation ( Supplementary Fig. S7 ). Again, the mean biodiversity richness per PU increased with connectivity in some cases, but the biodiversity at landscape scale decreased with higher connectivity; therefore, while more species per PU might have been included in the highest-ranked sites of higher connectivity, fewer unique species were conserved across the landscape. Maps with the highest connectivity measures were uninformative ( Supplementary Fig. S6 ). Overall, including connectivity in analyses served to further highlight the previously mentioned regions where C-stocking potential would also benefit biodiversity and ecosystem services while taking socioeconomic factors into consideration ( Fig. 2 , Supplementary Fig. S6 ). It is well established that Africa has great potential for C offset projects by reforestation [1] , [9] . There is, however, a need to pinpoint areas that are predicted to produce particularly high returns through C stocking by reforestation and avoid unintended costs and reap additional benefits for local communities, biodiversity conservation and other beneficiaries: knowledge that would be invaluable for estimating the benefits of C projects before their establishment [1] , [9] . Our investigation fills a major knowledge gap by producing the first map of C-stocking potential by reforestation for tropical Africa, or any other similarly large region, and indicating where such reforestation projects would provide substantial co-benefits. We identified areas where high productivity and high landscape disturbance or degradation overlap, and where C-stocking projects would thus bring high returns ( Figs 1 , 2 ), notably the Upper and Lower Guinean rainforests, the regions surrounding the Congolian rainforests and the shores of Lake Victoria. These all occur in the equatorial belt areas with high rainfall and warm temperatures, and thus high potential productivity, but have been subjected to considerable degradation [22] , [23] , [24] , [25] . In contrast, much of the Congolian rainforests, which also receive high rainfall, exhibited relatively low levels of C-stocking potential due to their comparatively low levels of degradation [24] , while the Sahel’s low potential for C stocking could be attributed to its low rainfall. There have been several calls to consider biodiversity, ecosystem services and socioeconomic factors in the planning of carbon offset projects [9] , [11] , [26] . Several studies have included existing C biomass as one of several factors that should be considered as a trade-off for identifying site conservation purposes or under the Reducing Emissions from Deforestation and Forest Degradation (REDD) scheme [27] , [28] , [29] , [30] ; however, there is a lack of concomitant information on how C stocking by forestation or forest restoration, that is, potential C biomass, could be traded off with such co-benefits. We assess where C-stocking projects should be placed to optimize positive synergies with other factors such as species conservation, ecosystem services and socioeconomic factors ( Fig. 2c , yellow areas). Generally, highly ranked areas when co-benefits were considered were similar to areas identified solely on the basis of C-stocking potential ( Fig. 2 , Supplementary Fig. S4 ). However, there were moderate shifts in geographic emphasis when co-benefits were considered. More extensive regions of the Upper and Lower Guinean rainforests were highly ranked; these regions thus not only have high C-stocking potential but also higher degrees of governance and levels of biodiversity ( Supplementary Fig. S8 ). They support several restricted-range species [31] , [32] but have, especially in West Africa, been extensively degraded, resulting in extensive local losses of forest species [23] , [33] , [34] . The Batéké Plateau was also identified as a high priority area, as it possesses high groundwater recharge, low land value and a relatively high governance index ( Supplementary Fig. S8 ). The Batéké Plateau is an extensive mosaic of savanna and gallery forests, some heavily degraded, stretching across central Congo (Brazaville) with a climate suitable for extensive forests [35] . Debate exists as to whether the savannas in this area are secondary [36] or whether they reflect earlier Holocene climate change [35] . Therefore, while reforestation in the region is possible, given the uncertainty of the ‘natural’ state of the savanna vegetation, specifically selecting recently degraded areas for reforestation would be advantageous. An area that was identified as having high C-stocking potential, but became less highly ranked when other factors were considered, is the region around Lake Victoria. It has seen a human population explosion since the 1930s due to improved accessibility and health conditions [22] , [37] , resulting in extensive deforestation and soil degradation [22] , [38] . Thus, while much of this region achieved top priority in terms of C-stocking potential alone, its high population density and intense agricultural productivity underlie substantial land values. The area also does not support particularly high terrestrial biodiversity ( Supplementary Fig. S8 ). Therefore, the region around Lake Victoria did not emerge as a top priority area when biodiversity, ecosystem services benefits and costs of C-stocking projects were also considered. Other regions of high C-stocking potential, but lower co-benefits, were several pockets North and South of the Congolian rainforest. Despite their high C-stocking potential, these regions tend to have low governance and do not support exceptional levels of biodiversity ( Supplementary Fig. S8 ). The latter can probably be attributed to past climate changes, which are thought to have resulted in the extinction or range contractions of species that previously occurred here [39] , [40] . Identifying areas with high C-stocking potential (with or without co-benefits) constitutes only the first step in setting up C-stocking projects by reforestation and a number of considerations and uncertainties. Caution should be taken that C projects by reforestation should not extensively conflict with existing land uses such as agriculture, as loss of agricultural activity on land earmarked for C-stocking projects could result in leakage, where C stocking in one area results in agricultural increases—and therefore loss of C stocks—in other areas [13] . Also, for reforestation projects to succeed in developing countries, surrounding communities must obtain benefits from forests and be actively involved in their management [41] , [42] . A number of co-benefits have been shown to improve the success of C-stocking projects. These include improved livelihoods that address local needs, increased incomes, the creation of employment opportunities and markets for, for example, non-timer forest products that could be harvested from within the reforested patch [41] . Future climate change comprises a further consideration for reforestation projects. Trees are long-lived organisms. The success of reforestation projects, and the ability of reforested areas to build up and maintain their C stocks may be influenced by whether and how climate change will affect the ability of plants to grow in novel climates [43] ; the African tropics may be especially prone to such effects [43] . Some of the areas under consideration in this study are likely to experience climates not currently experienced anywhere on Earth [43] , making it difficult to predict climate change effects. In addition, future climate change predictions for these areas have high uncertainty [44] , further complicating predictions of climate change effects on the vegetation and species of the region. Increases in atmospheric CO 2 are a further factor—they are likely to benefit tree growth due to CO 2 fertilization effects [45] , allowing even higher tree biomass, and thus C biomass, than predicted from our models to be sequestered in C-stocking forests. Finally, a number of uncertainties in analyses such as ours inevitably exist. These may, for example, arise due to the large scale at which the project was conducted, which brings about uncertainties in the input data that have usually been generated by a form of interpolation and/or on the basis of indirect remote sensing data. In addition, C-stocking potential may be affected by factors other than those that we used in our analyses, but might be difficult to obtain at large spatial scales, or might only act locally. The identification of potential sites for C stocking by forestation using methods such as ours should thus only serve as a first step in planning the location of potential sites. Subsequently integrating a wide range of expertise in site assessment, project identification, planning and execution is essential for ensuring the wider benefits of such projects. This integration would empower the description of existing ecological and socioeconomic conditions and promote the development of a detailed strategy that not only maximizes C-stocking potential but also considers ecosystem processes and features, cultural, monetary and managerial constraints and could examine uncertainties at a local level. In conclusion, the primary aim of C offset projects is to reduce atmospheric CO 2 concentrations. Although biodiversity and other ecosystem services often indirectly benefit from C-stocking projects [46] , policies that promote C stocking do not always benefit conservation or ecosystem services, nor is it always realistic to establish projects in areas with the highest C-stocking potential. Strategies that solely benefit C stocking may compromise biodiversity and water supply [30] , [47] , [48] , come at the expense of agricultural production [13] , negatively impact ecosystems [47] , [48] and local people [49] , or have costs associated with high land value or poor governance. Therefore, much can be gained if the planning of C projects considers co-benefits, costs and risks. Here, we demonstrate how prioritization of C projects can integrate factors beyond C stocking, including biodiversity conservation, ecosystem services and political and socioeconomic risks and costs. Consideration of these factors may influence geographic priorities and serve as a useful initial decision-making tool to balance various factors to maximize the overall benefits of C offset projects. Our site selection methods identify areas that should specifically benefit from restorative reforestation, for example, by planting a complement of woody species indigenous to the area, while the indigenous fauna are allowed to persist or are reintroduced. Setting aside landscapes for C-stocking purposes can make important contributions to mitigating climate change. If the selection of such landscapes is performed within a broader framework, stocking projects may also optimize wider benefits [50] . Assessing C-stocking potential This study focused on the potential of reforestation for C stocking. Because of data limitations (C estimates for non-woody vegetation, below-ground C and soil C are more difficult to attain [3] ), we assessed the potential for C storage in terms of aboveground woody biomass (henceforth ‘biomass’). Two maps of biomass for tropical Africa were used, one by Saatchi et al. [16] and the other by Baccini et al. [17] ( Fig. 1 , Supplementary Table S1 , Supplementary Methods ) [16] , [17] . The two maps are highly correlated ( Supplementary Table S5 ). Main analyses were run using both data sets; however, we mainly represent the results from the more recent map by Saatchi et al. [16] . We quantified the maximum C biomass that could be stored per unit area using two methods: (1) 90th-percentile QR and (2) OLS regressions ( Supplementary Methods ). Biomass was used as a response variable and modelled in terms of four climatic variables [51] that are important for the distribution of vegetation types across Africa [52] , and two soil variables [53] ( Supplementary Methods ). Confidence of model estimates was assessed, and the predicted maximum C biomass compared with aboveground C biomass measured in undisturbed forests across tropical Africa ( Supplementary Methods ). Two sets of maps of the difference between potential and actual C storage were created by subtracting the original biomass maps [16] , [17] from the maximum biomass calculated by QR and OLS. The resulting maps (‘C-stocking potential’ maps) represent alternative representations of the amount of biomass that each PU (that is, raster grid-cell) should be able to support under optimal conditions (no disturbances such as forest clearing or fire that could reduce woody biomass). The values of PUs with negative C-stocking potential (that is, where predicted maximum C-stocking potential was lower than the C biomass of original biomass maps) were changed to zero—this was 11% (QR) and 33% (OLS) of PUs in Saatchi analyses and 6% (QR) and 26% (OLS) in Baccini analyses. Carbon-stocking potential maps produced using 90% QR and OLS, based on both the Saatchi and Baccini data, were compared using Pearson’s product-moment correlation analyses. We chose to run QR models using 90% quantiles to prevent models from overestimating potential carbon storage. However, to ensure that running the analyses using higher quantiles would not result in different patterns of projected C-stocking potential, QR analyses were repeated using 98% quantiles ( Supplementary Methods ). These results are referred to in the supplement; except if otherwise stated, ‘QR’ here refers to 90% quantile regressions. Maps of C-stocking potential that were produced using 90 and 98% QR were also compared using Pearson’s correlation analyses. Selecting regions for C stocking We used the spatial prioritization technique Zonation [54] version 3.1.2 to select areas where C-stocking potential could be optimized while also maximizing conservation potential, an ecosystem service, and considering socioeconomic factors. Zonation identifies areas of high conservation priority by iteratively removing PUs that contribute least to the conservation targets from the full landscape, while taking other specified cost factors into consideration [55] . Analyses were run at a 10-km resolution ( Supplementary Methods ). Zonation analyses were mainly run using the ABF cell removal rule, although for comparative purposes analyses were repeated using the BCZ cell removal technique [54] ( Supplementary Methods ). Optimal areas for C-stocking projects were selected based on the occurrence and abundance of a number of features: C-stocking potential, biodiversity richness, groundwater recharge, governance and land value ( Supplementary Fig. S8 ). PUs with higher values for these features (lower values for land value), and complementarity to previously chosen features for species, had a higher probability of being selected. Species distribution and richness are perhaps the most basic, but also of the most important measures of diversity, and they constitute an important measure of conservation importance [56] . Therefore, as representatives of biodiversity features, distribution maps for all species of mammals, reptiles and amphibians were obtained from the IUCN [31] and included in analyses as separate layers. (A total of 979 mammals, 142 reptiles and 671 reptiles were recorded for the region). We used species distributions rather than species richness maps, as this allowed PUs to be selected on both the number and rarity of their species [54] . Groundwater recharge, the amount of water that filters from the earth’s surface to replenish groundwater supplies, is an important ecosystem service [57] . Since groundwater is protected from surface pollution and experiences less fluctuation in levels than surface water sources, lack of groundwater recharge can limit sustainable groundwater usage [57] . Therefore, a map of groundwater recharge [57] was used as a feature layer in our analyses. Areas with high groundwater recharge were considered to be of high value. Socioeconomic factors were also included as features in our analysis. Land cost is a constraining factor in setting aside land for C stocking. Although prices for C credits vary widely between projects, it is essential that the benefits of stocking are profitable [12] . Naidoo and Iwamura [58] mapped global land value as a function of crop productivity, livestock density and consumer prices of crops and livestock to calculate gross economic rents of the land. In addition to land value, this index is also representative of agricultural productivity. Land value was included in our assessment with negative weighting, that is, areas with low land value were preferentially selected. Governance is essential to ensure that incentives with co-benefits for communities or biodiversity are successful [59] , as the lack of capacity to manage and ensure the success of such incentives may lead to their failure. Therefore, PUs were positively selected if they were associated with a higher Ibrahim Index of African Governance [60] . This index is produced on national scale as a function of four categories: safety and rule of law, participation and human rights, sustainable economic opportunity and human development [60] . Including this index in our site selection process did not mean that areas with poor governance would not be selected; however, a higher cost was associated with poor governance. Landscapes unsuitable for C-stocking projects were excluded from analyses ( Supplementary Methods ). Features can be weighted differently in Zonation analyses so that some features are prioritized over others. Here, all features were equally weighted [27] : groundwater recharge and governance received a weighting of three, and land value weighted negative three. For species richness, each taxonomic group carried a weight of one so that the final weight carried by faunal biodiversity also summed to three. Each species was weighted as a function of the number of species in their taxonomic class in the region considered here [27] , with each mammal species weighted at 1/979, reptile species at 1/142 and amphibian species at 1/671. Finally, since we focused on C-stocking potential, its weight was varied in separate runs (weights of 3, 6, 12, 24 and 48). These weightings reflect different prioritizations of C-stocking potential, ranging from being equal to each of the other factors, to being assigned four times the weight of the other factors combined. For comparative purposes, Zonation models were run where only C-stocking potential was included as a feature. This analysis identified the PUs that would be selected based on C-stocking potential alone. All these prioritization runs thus span strategies in which C stocking is considered as one of several equally important factors in landscape planning to strategies in which C stocking is the primary goal. The output of prioritization maps included maps ranking each PU in terms of the features and their weightings that were specified in the analyses. Highest-ranked PUs were most favourable for the conditions that were specified during the prioritization runs. The performance trade-offs of using different weightings for C-stocking potential were calculated for the top 5% highest-ranked PUs and for all PUs ( Supplementary Methods ). In addition, two-tailed Spearman rank correlation was used to compare different prioritization runs, that is, the order in which PUs were removed during Zonation analyses for different cell removal methods and different data sets ( Supplementary Methods ). Finally, Zonation analyses where connectivity of sites was accounted for [55] were run using different boundary length parameters ( Supplementary Methods ). Increasing connectivity among sites reduces fragmentation of high priority sites in the landscape, and thus identifies larger contiguous regions where carbon sequestration would be beneficial considering the other features taken into account here. An outline of which of the two C data sets were used for which combination of analyses to calculate C-stocking potential and to create maps of the trade-off between C stocking potential and other factors are presented in Supplementary Table S1 . How to cite this article: Greve, M. et al. Spatial optimization of carbon-stocking projects across Africa integrating stocking potential with co-benefits and feasibility. Nat. Commun. 4:2975 doi: 10.1038/ncomms3975 (2013).